Reversible inactivation of deubiquitinases by reactive oxygen speciesin vitroand in cells In eukaryotes, deubiquitinases (DUBs) remove ubiquitin conjugates from diverse substrates, altering their stabilities, localizations or activities. Here we show that many DUBs of the USP and UCH subfamilies can be reversibly inactivated upon oxidation by reactive oxygen species in vitro and in cells. Oxidation occurs preferentially on the catalytic cysteine, abrogating the isopeptide-cleaving activity without affecting these enzymes’ affinity to ubiquitin. Sensitivity to oxidative inhibition is associated with DUB activation wherein the active site cysteine is converted to a deprotonated state prone to oxidation. We demonstrate that this redox regulation is essential for mono-ubiquitination of proliferating-cell nuclear antigen in response to oxidative DNA damage, which initiates a DNA damage-tolerance programme. These findings establish a novel mechanism of DUB regulation that may be integrated with other redox-dependent signalling circuits to govern cellular adaptation to oxidative stress, a process intimately linked to aging and cancer. Ubiquitination is a widespread posttranslational modification that controls many essential cellular processes in eukaryotes [1] , [2] . Once conjugated to substrates, ubiquitin can be removed by a family of isopeptidases termed deubiquitinases (DUB), which reverse the function of ubiquitination. In addition, deubiquitination allows ubiquitin to be recycled [3] , [4] . The human genome encodes ∼ 100 DUBs that belong to five subfamilies. The largest group is the USP subfamily with 56 members that each has a conserved USP domain. Another important class is the UCH family, which has four members. All DUBs, except for those in the JAMM subfamily (12 in human), are cysteine proteases whose activities are dependent on an active site cysteine residue. This catalytic cysteine is situated in a cleft proximal to a His and an Asp residue, forming a triad that lowers the pKa of the catalytic cysteine during catalysis [5] , [6] . To date, many important cellular factors have been identified as DUB substrates, including p53, TRAF2, FANCD2 and proliferating-cell nuclear antigen (PCNA) [7] , [8] , [9] , [10] . By acting on diverse substrates, DUBs can have enormous influence on cell physiology. Accordingly, mutations in DUBs have been linked to many human diseases including cancer and Parkinson’s disease [11] , [12] , [13] , [14] . Reactive oxygen species (ROS), such as superoxide (O2 − ), hydrogen peroxide (H 2 O 2 ) and hydroxyl radical (HO·), are by-products of mitochondrial oxidative metabolism, constantly produced in eukaryotic cells [15] . When certain metabolic pathways are deregulated, the levels of intracellular ROS can be elevated to surpass the cellular antioxidant capacity, resulting in oxidative stress. ROS are known for their damaging effects on nucleic acids, cellular enzymes and lipids. Accordingly, oxidative stress is widely associated with various human diseases, such as cancer, Alzheimer’s disease and aging [16] , [17] , [18] . However, accumulating evidence also suggests that ROS, particularly endogenous H 2 O 2 , can have important physiological functions in regulating redox-dependent signalling outputs and pathogen–host interactions [19] , [20] . For example, H 2 O 2 produced in phagocytic cells in response to microbial invasion can serve a direct anti-microbial function when it attacks the DNA and proteins of pathogens [21] . Another well-characterized example is a group of protein tyrosine phosphatases (PTPs) whose catalytic cysteines are prone to oxidation, which reversibly inactivates these enzymes [22] , [23] , [24] . In this study, we demonstrate that DUBs can be reversibly inhibited by exogenously and endogenously produced ROS due to oxidation of the catalytic cysteine, a reaction prone to occur while the DUB active site undergoes deprotonation during activation. We further show that DUB inhibition is essential for mono-ubiquitination of PCNA in cells encountering oxidative stress, which is known to activate the translesion synthesis (TLS) pathway in order to maintain DNA replication in stressed cells. Redox-dependent regulation of DUBs in vitro We expressed and purified 34 DUBs ( ∼ 1/3 of the human DUBs), each as a FLAG-tagged protein from HEK293 cells ( Supplementary Fig. S1 ). Most of these DUBs (25) belong to the USP subfamily, with the exception of UCH-L1, UCH-L3, UCH-L5 and BAP1, which belong to the UCH subfamily, and YOD1, A20, VCPIP1 and OTUD7B, which are in the OTU subfamily, and JOSD2, a Josephin subfamily member [5] . We measured the activity of each DUB in vitro using ubiquitin-7-amino-4-trifluoromethylcoumarin (AFC) (Ub-AFC) as the substrate, as cleavage of the AFC group by the DUBs generates fluorescence [25] . Interestingly, most DUBs analysed did not show any significant activities ( Fig. 1a–c ). Serendipitously, we found that incubation of many DUBs with the thiol-reducing agent dithiothreitol (DTT) activated them ( Fig. 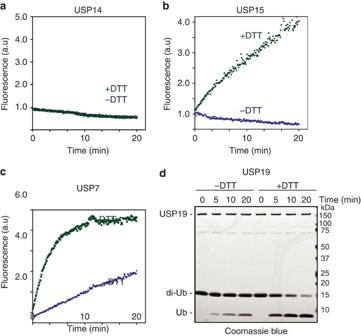Figure 1: Redox-dependent regulation of DUBs. (a–c) Activation of DUBsin vitro. Shown are representative DUB activity curves. Purified DUBs were incubated with Ub-AFC and the fluorescence intensities were recorded as a function of time. Where indicated, the DUBs were pretreated with 1 mM DTT for 10 min. (d) DTT activates USP19. Purified USP19 was treated with or without 1 mM DTT for 10 min before incubated with Lys48-linked di-ubiquitin. The DUB activity was measured by SDS–PAGE analysis. 1a–c , Table 1 ). This could be further demonstrated using Lys48-linked diubiquitin as the substrate ( Fig. 1d ). Based on our results ( Table 1 ), we grouped these DUBs into three categories. The first group had no activity regardless of whether or not DTT was present. The DUBs in the second group had little activity by themselves, but significant activity could be detected after DTT treatment. The DUBs in the third class were active by themselves, but the activity could be further enhanced by DTT. Figure 1: Redox-dependent regulation of DUBs. ( a – c ) Activation of DUBs in vitro . Shown are representative DUB activity curves. Purified DUBs were incubated with Ub-AFC and the fluorescence intensities were recorded as a function of time. Where indicated, the DUBs were pretreated with 1 mM DTT for 10 min. ( d ) DTT activates USP19. Purified USP19 was treated with or without 1 mM DTT for 10 min before incubated with Lys48-linked di-ubiquitin. The DUB activity was measured by SDS–PAGE analysis. Full size image Table 1 The effects of DTT on deubiquitinases. Full size table Our results immediately suggested that DUBs might be subject to regulations by redox state, as the lack of activity in our initial experiments could be due to oxidation during purification. To test this idea, we used USP19, a membrane-associated DUB implicated in endoplasmic reticulum (ER)-associated degradation [26] , [27] , as a model because it could be purified from HEK293 cells in large quantity. We first measured the effect of H 2 O 2 , a ROS commonly produced in humans, on USP19. The results showed that USP19 purified under reducing conditions readily cleaved either Ub-AFC or Lys48-linked diubiquitin, but upon treatment with H 2 O 2 , its activity was completely abolished ( Fig. 2a ). As expected, this inhibition was reversed by DTT ( Fig. 2b ). 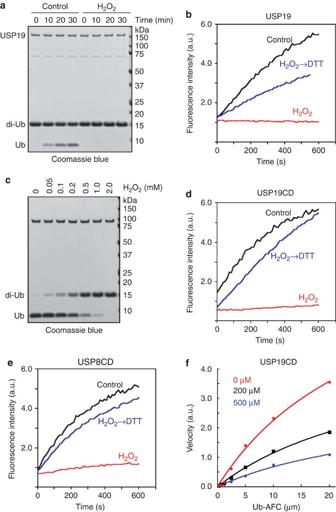Figure 2: Inhibition of DUBs by H2O2. (a,b) Inhibition of USP19 by H2O2. USP19 purified under reducing conditions was treated with 0.5 mM H2O2for 3 min and the DUB activity was assayed using either di-ubiquitin (a) or Ub-AFC (b) as the substrate. Where indicated, H2O2-treated USP19 (200 nM) was subsequently incubated with 2 mM DTT before the analysis. (c,d) The catalytic domain (CD) of USP19 is sensitive to inactivation by H2O2. (c) Di-ubiquitin was treated with USP19CD in the presence of the indicated concentrations of H2O2. (d), As inb, except that USP19CD (50 nM) was used.Note: The di-ubiquitin cleavage assay was performed in a smaller volume (20 μl) than the Ub-AFC assay (200 μl). Thus, more DTT was carried over by the enzyme. (e) The activity of USP8CD is reversibly inactivated by H2O2. (f) Oxidation significantly reduces the catalysis constant (Kcat) of USP19CD. USP19CD pretreated with 0, 200 or 500 μM H2O2was incubated with the indicated concentrations of Ub-AFC. The DUB activities measured under each substrate concentration were plotted. Figure 2: Inhibition of DUBs by H 2 O 2 . ( a , b ) Inhibition of USP19 by H 2 O 2 . USP19 purified under reducing conditions was treated with 0.5 mM H 2 O 2 for 3 min and the DUB activity was assayed using either di-ubiquitin ( a ) or Ub-AFC ( b ) as the substrate. Where indicated, H 2 O 2 -treated USP19 (200 nM) was subsequently incubated with 2 mM DTT before the analysis. ( c , d ) The catalytic domain (CD) of USP19 is sensitive to inactivation by H 2 O 2 . ( c ) Di-ubiquitin was treated with USP19CD in the presence of the indicated concentrations of H 2 O 2 . ( d ), As in b , except that USP19CD (50 nM) was used. Note : The di-ubiquitin cleavage assay was performed in a smaller volume (20 μl) than the Ub-AFC assay (200 μl). Thus, more DTT was carried over by the enzyme. ( e ) The activity of USP8CD is reversibly inactivated by H 2 O 2 . ( f ) Oxidation significantly reduces the catalysis constant ( K cat ) of USP19CD. USP19CD pretreated with 0, 200 or 500 μM H 2 O 2 was incubated with the indicated concentrations of Ub-AFC. The DUB activities measured under each substrate concentration were plotted. Full size image USP19 contains several regulatory domains in addition to the conserved USP domain that harbours the catalytic triad residues Cys506, His1165 and Asp1189. To see whether H 2 O 2 inhibits USP19 by acting through the catalytic domain, we expressed and purified the USP domain of USP19 (USP19CD). Purified USP19CD behaved similarly to full-length USP19 as it contained little activity unless treated with DTT ( Supplementary Fig. S2 ). Exposure of USP19CD to H 2 O 2 strongly inhibited its activity, which was abolished by DTT ( Fig. 2c ). Similar results were obtained with the catalytic domain of USP8 ( Fig. 2e ), suggesting that DUBs can be reversibly inactivated by oxidation of a cysteine residue(s) in the catalytic domain. The catalytic cysteines of DUBs are prone to oxidization We next measured the effect of substrate concentration on H 2 O 2 -mediated inhibition using USP19CD. Fitting the calculated velocity data with Michaelis–Menten kinetics revealed that H 2 O 2 treatment significantly reduced the catalytic constant K cat without affecting the K m value, indicating that oxidation alters the DUBs’ capability to cleave ubiquitin isopeptide bonds without affecting their affinity to ubiquitin ( Fig. 2f ). Thus, the target of ROS may be the catalytic core. It is known that oxidation often occurs on cysteine that can overcome the high pKa ( ∼ 8.5) at the physiological pH. This requires another amino acid to serve as a base that lowers the cysteine pKa. Therefore, the catalytic cysteine in DUBs is an ideal target of ROS, because the other residues in the catalytic triad usually facilitate the deprotonation of this cysteine during activation. To test whether ROS targets the DUB active site cysteine, we treated wild-type (WT) USP19CD and a catalytically inactive mutant bearing the C506S substitution with H 2 O 2 . Electrophoresis under non-reducing conditions showed that a significant fraction of WT USP19CD migrated more slowly upon treatment with H 2 O 2 (indicated by the asterisk in Fig. 3a ), apparently due to oxidation. In addition, a small fraction of USP19CD formed disulphide-linked oligomers (arrowhead in Fig. 3a ). As expected, these oxidized USP19 species were abolished under reducing electrophoresis conditions (lanes 9–12), and were not detected for USP19CD C506S (lanes 5–8, 13–16), demonstrating that the catalytic cysteine is required for efficient oxidation. 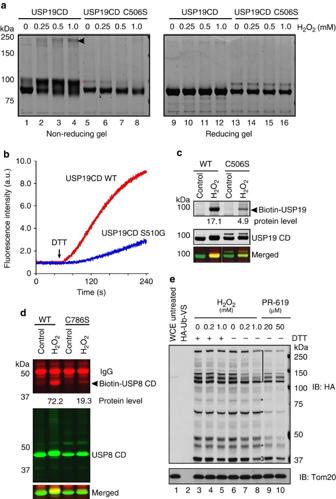Figure 3: The catalytic cysteines in DUBs are prone to oxidationin vitroandin vivo. (a) Reversible oxidation of the catalytic cysteine of USP19. Purified USP19CD WT or C506S was treated with the indicated concentrations of H2O2for 10 min then analysed by either non-reducing or reducing SDS–PAGE electrophoresis. Asterisk indicates an oxidized species. The arrowhead indicated band likely represents disulphide-linked USP19 oligomer. (b) Ser510 in USP19 is required for the reversibility of the redox regulation. Equal amount of USP19CD WT and the S510G mutant treated with 0.5 mM H2O2were assayed for DUB activity. Where indicated, DTT (1 mM) was added. (c,d) The catalytic cysteine of DUBs is preferentially oxidized by H2O2in vivo. HEK293 cells transfected with plasmids expressing either USP19CD (c) or USP8CD (d) were treated with 1 mM H2O2for 5 min followed by biotin labelling. The numbers indicate the relative levels of biotin-labelled DUBs. (e) H2O2inhibits the labelling of endogenous DUBs by HA-tagged ubiquitin vinyl sulphone (HA-Ub-VS). Cells treated with either H2O2or the DUB inhibitor PR-619 were incubated for 10 min at 37 °C in a labelling buffer containing 0.5% NP40 and HA-Ub-VS (2 μM). Where indicated, the buffer also contained 5 mM DTT. The whole-cell extracts were analysed by immunoblotting (IB). The brackets indicate DUBs that are sensitive to H2O2. A few Ub-VS reactive DUBs appear to be insensitive to H2O2(indicated by asterisks), probably because their active sites are not organized unless treated with HA-Ub-VS. At this point, H2O2has been removed. Whole cell extract (WCE). Figure 3: The catalytic cysteines in DUBs are prone to oxidation in vitro and in vivo . ( a ) Reversible oxidation of the catalytic cysteine of USP19. Purified USP19CD WT or C506S was treated with the indicated concentrations of H 2 O 2 for 10 min then analysed by either non-reducing or reducing SDS–PAGE electrophoresis. Asterisk indicates an oxidized species. The arrowhead indicated band likely represents disulphide-linked USP19 oligomer. ( b ) Ser510 in USP19 is required for the reversibility of the redox regulation. Equal amount of USP19CD WT and the S510G mutant treated with 0.5 mM H 2 O 2 were assayed for DUB activity. Where indicated, DTT (1 mM) was added. ( c , d ) The catalytic cysteine of DUBs is preferentially oxidized by H 2 O 2 in vivo . HEK293 cells transfected with plasmids expressing either USP19CD ( c ) or USP8CD ( d ) were treated with 1 mM H 2 O 2 for 5 min followed by biotin labelling. The numbers indicate the relative levels of biotin-labelled DUBs. ( e ) H 2 O 2 inhibits the labelling of endogenous DUBs by HA-tagged ubiquitin vinyl sulphone (HA-Ub-VS). Cells treated with either H 2 O 2 or the DUB inhibitor PR-619 were incubated for 10 min at 37 °C in a labelling buffer containing 0.5% NP40 and HA-Ub-VS (2 μM). Where indicated, the buffer also contained 5 mM DTT. The whole-cell extracts were analysed by immunoblotting (IB). The brackets indicate DUBs that are sensitive to H 2 O 2 . A few Ub-VS reactive DUBs appear to be insensitive to H 2 O 2 (indicated by asterisks), probably because their active sites are not organized unless treated with HA-Ub-VS. At this point, H 2 O 2 has been removed. Whole cell extract (WCE). Full size image To understand the chemical nature of ROS-induced modification, we excised the oxidized USP19CD from the gel and analysed it by mass spectrometry. The experiment identified a catalytic cysteine-containing peptide that carried a sulphenyl-amide intermediate at the cysteine residue ( Supplementary Fig. S3a,b ). Because it was demonstrated that for PTPs, the formation of a sulphenyl-amide intermediate requires a serine residue adjacent to the active site cysteine [22] , we used a USP19CD structural model obtained by homology modelling (Lee, J. unpublished results) to identify a serine residue (Ser510) that is near the active site. We created and purified the USP19CD S510G mutant. Similar to WT USP19CD, the S510G mutant had activity that was sensitive to ROS ( Supplementary Fig. S4a ; Fig. 3b ). However, once inactivated by H 2 O 2 , DTT could not effectively restore the activity of USP19CD S510G ( Fig. 3b ). These results suggest that Ser510 may be involved in the formation of a sulphenyl-amide intermediate, which maintains USP19 in an inactive but reactivable state. The conservation of this serine residue in many DUBs ( Supplementary Fig. S4b ) raises the possibility that our finding may be applicable to other ROS-sensitive DUBs. That being said, our study cannot rule out the possibility that other forms of oxidation may also occur in USP19 or other DUBs. We next tested whether catalytic cysteines in DUBs are prone to oxidation in cells exposed to H 2 O 2 . We treated cells expressing either USP19CD or USP19CD C506S mutant with H 2 O 2 . Cell extracts were prepared in the presence of N -ethylmaleimide (NEM), which modified solvent-exposed cysteine residues except for those oxidized by H 2 O 2 . USP19 and the mutant protein immunoprecipitated from cell extracts were then incubated with DTT to reverse oxidation before being treated with a cysteine-reactive biotinylating reagent. Under these conditions, only cysteines oxidized by H 2 O 2 escape alkylation by NEM, and therefore, are biotinylated. Immunoblotting showed that WT USP19CD, but not the USP19CD C506S mutant, could be biotinylated efficiently in a H 2 O 2 -dependent manner ( Fig. 3c , Supplementary Fig. S4c ). Similar observation was obtained with USP8CD ( Fig. 3d ). These results indicate that the catalytic cysteine of these DUBs is preferentially oxidized by H 2 O 2 in cells. To determine whether oxidation occurs on the active site of endogenous DUBs in oxidatively stressed cells, we lysed untreated or H 2 O 2 -treated cells in a buffer containing haemagglutinin (HA)-tagged ubiquitin vinyl sulphone (HA-Ub-VS), an active site-directed inhibitor. Immunoblotting showed that H 2 O 2 treatment causes a decrease in Ub-VS-labelled DUBs ( Fig. 3e , lanes 7, 8 versus lane 6), suggesting that H 2 O 2 converted the active site of endogenous DUBs to a state not reactive to Ub-VS. Importantly, addition of DTT to the lysis buffer restored Ub-VS-labelling signals (lanes 3–5). As a positive control, we treated cells with the reversible DUB inhibitor, PR-619. As expected, when the active sites were competitively blocked, the Ub-VS-labelling efficiency was significantly reduced (lanes 9, 10). Although the Ub-VS-labelling experiment cannot rule out the possibility of an allosteric effect, the results are in accordance with our in vitro studies, suggesting that the catalytic cysteines of DUBs are prone to oxidation by ROS. Sensitivity to ROS is associated with DUB activation The observation that some DUBs purified in the absence of any reducing agents (group 3) still contain significant activities suggests that these DUBs might be more resistant to inhibition by ROS than those that had lost their activity during purification (group 2). We therefore chose USP19 as a representative for group 2, USP7 and UCH-L1 for group 3 ( Fig. 4a ), and compared the effect of H 2 O 2 on the activities of these enzymes. Consistent with our hypothesis, both USP19 and USP19CD were highly sensitive to H 2 O 2 ( Fig. 4b ). By contrast, USP7 and UCH-L1 were more resistant to H 2 O 2 -mediated inhibition at pH 7.4 ( Fig. 4c ). 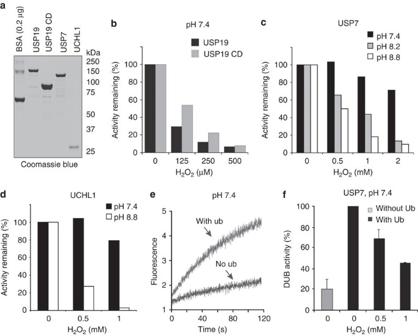Figure 4: Sensitivity to oxidative inhibition is associated with DUB activation. (a) Purified DUBs used in the assays. A known amount of BSA was used to estimate the concentration of the purified DUBs. (b) USP19 is highly sensitive to inhibition by H2O2. Purified USP19 or USP19CD was treated with the indicated concentrations of H2O2at pH 7.4. The samples were diluted tenfold before the DUB activities were determined by the Ub-AFC assay. (c,d) The sensitivity of USP7 and UCH-L1 to inhibition by H2O2is enhanced by high pH. USP7 or UCH-L1 was treated with H2O2at the indicated pH and the DUB activity was determined by the Ub-AFC assay. (e) Ubiquitin activates USP7. USP7 was incubated at pH 7.4 in the absence or presence of ubiquitin (50 μM). The samples were diluted tenfold before Ub-AFC was added to determine the USP7 activities. (f) USP7 activation by ubiquitin sensitizes it to inhibition by H2O2. USP7 was pretreated in a buffer without or with ubiquitin for 5 min. Where indicated, H2O2was also included. The USP7 activities were determined by the Ub-AFC assay at pH 7.4. The error bars indicate the mean of two independent experiments. Figure 4: Sensitivity to oxidative inhibition is associated with DUB activation. ( a ) Purified DUBs used in the assays. A known amount of BSA was used to estimate the concentration of the purified DUBs. ( b ) USP19 is highly sensitive to inhibition by H 2 O 2 . Purified USP19 or USP19CD was treated with the indicated concentrations of H 2 O 2 at pH 7.4. The samples were diluted tenfold before the DUB activities were determined by the Ub-AFC assay. ( c , d ) The sensitivity of USP7 and UCH-L1 to inhibition by H 2 O 2 is enhanced by high pH. USP7 or UCH-L1 was treated with H 2 O 2 at the indicated pH and the DUB activity was determined by the Ub-AFC assay. ( e ) Ubiquitin activates USP7. USP7 was incubated at pH 7.4 in the absence or presence of ubiquitin (50 μM). The samples were diluted tenfold before Ub-AFC was added to determine the USP7 activities. ( f ) USP7 activation by ubiquitin sensitizes it to inhibition by H 2 O 2 . USP7 was pretreated in a buffer without or with ubiquitin for 5 min. Where indicated, H 2 O 2 was also included. The USP7 activities were determined by the Ub-AFC assay at pH 7.4. The error bars indicate the mean of two independent experiments. Full size image Because oxidation preferentially occurs on deprotonated cysteine, the differential sensitivity to ROS might be due to differences in the active sites of these DUBs. USP19 may be constitutively activated, which enables deprotonation of the catalytic cysteine at the physiological pH. By contrast, USP7 is known to contain a disordered active site unless bound to the substrate/cofactors [28] . If sensitivity to oxidation is mechanistically linked to DUB activation, which requires deprotonation of the catalytic cysteines, increasing pH should enhance the sensitivity to ROS because high pH can activate many DUBs including USP7 and UCHs by facilitating cysteine deprotonation [29] , [30] . Indeed, H 2 O 2 had a much stronger inhibitory effect on USP7 at pH 8.2 or 8.8 than at pH 7.4 ( Fig. 4c ). Likewise, UCH-L1 also became highly sensitive to inhibition by H 2 O 2 at pH 8.8 ( Fig. 4d ). To further demonstrate the link between DUB activation and the sensitivity to ROS, we seek an alternative method to activate USP7. We found that similar to USP5 (ref. 31 ), pre-incubation of USP7 with free ubiquitin containing an unmodified carboxy terminus stimulated its activity by approximately fivefold ( Fig. 4e ). Ubiquitin may bind the ‘switching loop’ or potentiate the interaction between the ‘switching loop’ and the C-terminal ubiquitin-like domains of USP7, resulting in enhanced substrate binding [29] . Interestingly, when USP7 was treated with H 2 O 2 in the presence of this allosteric activator, its sensitivity to ROS was increased similarly to that caused by high pH ( Fig. 4f ). We conclude that the sensitivity to oxidative inhibition is intimately associated with DUB activation during which deprotonation of the catalytic cysteine occurs. Oxidative stress inhibits DUBs in vivo We next tested whether DUBs are subject to regulation by oxidative stress in cells. We first used Ub-AFC to measure the DUB activity in whole-cell extracts prepared from either control or H 2 O 2 -treated cells. The results showed that a short treatment with H 2 O 2 resulted in ∼ 90% loss of the DUB activities in HEK293 cells, which could be restored by DTT treatment ( Fig. 5a ). By contrast, neither the ER stress inducers tunicamycin and thapsigargin nor the DNA damaging agents methyl methanesulfonate (MMS) and bleomycin affected the DUB activities ( Supplementary Fig. S5a,b ), suggesting that DUB inhibition by H 2 O 2 is not due to general cytotoxicity. Instead, it must be caused by changes in cellular redox state. Several lines of evidence further corroborated this idea. First, treating cell extracts in vitro with H 2 O 2 also inhibited DUBs in a reversible manner ( Fig. 5c ). In fact, DTT treatment consistently resulted in increased DUB activities compared with untreated control extracts, suggesting that moderate oxidation might have occurred to some DUBs during sample preparation even in the absence of H 2 O 2 . In addition, DUB inhibition by H 2 O 2 could be prevented by growing the cells in a medium containing the anti-oxidant N -acetyl cysteine (NAC; Supplementary Fig. S5c ). Finally, gel filtration analysis showed that the DUB activities in whole-cell extract were present in two peaks ( Supplementary Fig. S6 ). The major peak co-migrated with proteins of ∼ 30 kDa, consistent with the size of the UCH family DUBs. The other peak was generated by DUBs associated with large protein complexes. Both peaks could be inhibited by H 2 O 2 , suggesting that DUB inhibition by ROS occurs in a global manner. 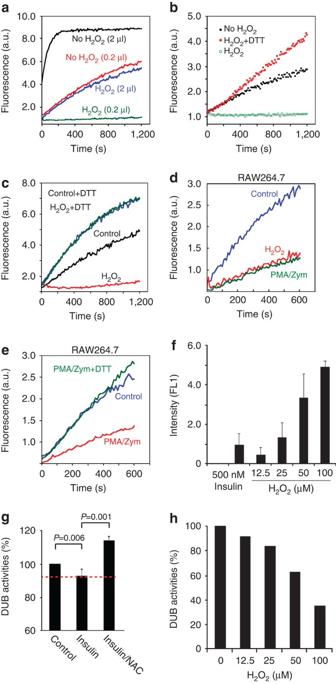Figure 5: Oxidative stress attenuates DUB activities in cells. (a) Treatment of HEK293 cells with H2O2resulted in the loss of DUB activity. HEK293 cells either untreated or treated with 1 mM H2O2for 30 min were lysed. The DUB activities in the indicated amount of whole-cell extracts were measured by the Ub-AFC assay. (b) DUB inhibition by oxidation is reversible. Where indicated, the extract of H2O2-treated cells was incubated with 1 mM DTT for 10 min before DUB activity was measured. (c) Inhibition of DUBs by H2O2in vitro. The whole-cell extracts prepared from HEK293 cells were either untreated or treated with 200 μM H2O2for 30 min. Where indicated, H2O2-treated extracts were further incubated with DTT before the DUB assay. (d–g) DUB activity was reversibly inhibited by endogenous ROS. (d) Whole-cell extracts were prepared from RAW264.7 cells treated with phorbol myristate acetate (PMA) plus Zymosan (Zym) (1 h). Untreated and H2O2-treated cells are controls. The DUB activity was measured as ina. (e), As in (d). Where indicated, 1 mM DTT was added to the extract of PMA/Zym-treated cells. (f) ROS generation was stimulated in HepG2 cells by insulin signalling. HepG2 cells treated with insulin (500 nM, 5 min) were stained with 10 μM DCFDA. Fluorescence intensity was measured by flow cytometry. Untreated cells were used to determine the background fluorescence. The error bars indicate the mean of two independent experiments. (g) Insulin signaling inhibits DUB activities in a redox-dependent manner. HepG2 cells treated with insulin or insulin together with NAC were lysed in a buffer containing Ub-AFC. The graph summarizes the results of five independent experiments (Error bars, standard deviation,n=5;P-values were calculated using paired Student’st-test). (h) Dose-dependent inhibition of DUB activities in HepG2 cells by H2O2. Figure 5: Oxidative stress attenuates DUB activities in cells. ( a ) Treatment of HEK293 cells with H 2 O 2 resulted in the loss of DUB activity. HEK293 cells either untreated or treated with 1 mM H 2 O 2 for 30 min were lysed. The DUB activities in the indicated amount of whole-cell extracts were measured by the Ub-AFC assay. ( b ) DUB inhibition by oxidation is reversible. Where indicated, the extract of H 2 O 2 -treated cells was incubated with 1 mM DTT for 10 min before DUB activity was measured. ( c ) Inhibition of DUBs by H 2 O 2 in vitro . The whole-cell extracts prepared from HEK293 cells were either untreated or treated with 200 μM H 2 O 2 for 30 min. Where indicated, H 2 O 2 -treated extracts were further incubated with DTT before the DUB assay. ( d – g ) DUB activity was reversibly inhibited by endogenous ROS. ( d ) Whole-cell extracts were prepared from RAW264.7 cells treated with phorbol myristate acetate (PMA) plus Zymosan (Zym) (1 h). Untreated and H 2 O 2 -treated cells are controls. The DUB activity was measured as in a . ( e ), As in ( d ). Where indicated, 1 mM DTT was added to the extract of PMA/Zym-treated cells. ( f ) ROS generation was stimulated in HepG2 cells by insulin signalling. HepG2 cells treated with insulin (500 nM, 5 min) were stained with 10 μM DCFDA. Fluorescence intensity was measured by flow cytometry. Untreated cells were used to determine the background fluorescence. The error bars indicate the mean of two independent experiments. ( g ) Insulin signaling inhibits DUB activities in a redox-dependent manner. HepG2 cells treated with insulin or insulin together with NAC were lysed in a buffer containing Ub-AFC. The graph summarizes the results of five independent experiments (Error bars, standard deviation, n =5; P -values were calculated using paired Student’s t -test). ( h ) Dose-dependent inhibition of DUB activities in HepG2 cells by H 2 O 2 . Full size image We next tested whether DUB inhibition takes place under physiological conditions of H 2 O 2 production. H 2 O 2 can be produced in cells by a family of nicotinamide adenine dinucleotide phosphate oxidases. Accordingly, the intracellular H 2 O 2 levels are significantly elevated in response to activation of certain signalling pathways or during oncogenic transformation [32] , [33] , [34] . A well-established system of endogenous H 2 O 2 production is the macrophage/monocyte cell line RAW264.7. Upon activation of Toll-like receptors (TLRs), the production of H 2 O 2 via nicotinamide adenine dinucleotide phosphate oxidase is strongly activated, as revealed by the fluorogenic ROS reporter 2′,7′-dichlorofluorescein diacetate (DCFDA) ( Supplementary Fig. S7 ) [35] , [36] . Using Ub-AFC as the substrate, we demonstrated that treatment of RAW264.7 cells with the TLR2 ligand Zymosan and the phorbol ester, phorbol myristate acetate, activators of the TLR pathways, inhibited endogenous DUBs similar to H 2 O 2 ( Fig. 5d ). As anticipated, this inhibition could be reversed by DTT ( Fig. 5e ). Endogenous H 2 O 2 is also generated during insulin signalling. It was shown that in both human adipocytes and a hepatoma cell line (HepG2) insulin treatment elicits a rapid burst of H 2 O 2 production [37] , [38] . DCFDA staining showed that the fluorescence intensity of insulin-treated HepG2 cells was comparable to that of cells treated with ∼ 20 μM H 2 O 2 ( Fig. 5f ). The Ub-AFC assays showed reproducibly that insulin-treated HepG2 cells contained reduced DUB activity ( Fig. 5g ), comparable to that in cells exposed to low concentrations of H 2 O 2 ( Fig. 5h ). Importantly, the DUB inhibition by insulin treatment was completely prevented by pre-treating cells with NAC ( Fig. 5g ). Together, these results indicate that both exogenous and endogenous H 2 O 2 can cause DUB inhibition in living cells. DUB inhibition accounts for PCNA monoubiquitination We next tested whether DUB inhibition upon oxidative stress could affect a physiologically relevant ubiquitination event in the cell. We investigated PCNA ubiquitination because this modification occurs in cells containing damaged DNA, and oxidative stress is a well-established inducer of DNA damage [8] , [39] . To this end, total cell extract prepared from cells exposed to H 2 O 2 was subject to immunoblotting with an antibody against PCNA. For a fraction of the cells (3,000 cells), we carried out a deubiquitinating assay by injecting the cells into a detergent-containing buffer that also contained Ub-AFC. Because cell lysis was coupled to the activity measurements, this protocol minimized the effect of oxidization during sample preparation. Our results showed that H 2 O 2 inhibited DUBs almost instantly upon treatment with H 2 O 2 , but over time, the DUB activities could be partially recovered, likely due to the launching of the cellular anti-oxidant programme ( Fig. 6a ). Immunoblotting showed that concurrent with DUB inhibition, ubiquitinated PCNA rapidly accumulated ( Fig. 6b ). A H 2 O 2 titration experiment showed that both ubiquitination of PCNA and DUB inhibition occurs in a H 2 O 2 concentration-dependent manner ( Supplementary Fig. S8a,b ). Thus, ubiquitination of PCNA correlates with DUB inhibition in oxidatively stressed cells. 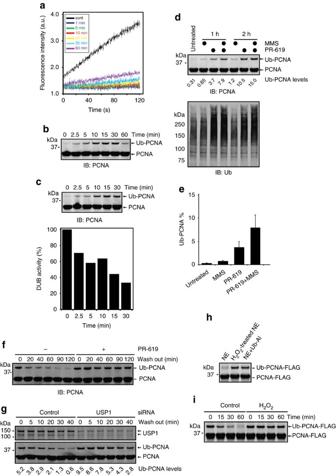Figure 6: DUB inhibition in oxidative-stressed cells facilitates PCNA ubiquitination. (a) The kinetics of DUB inhibition by H2O2. H2O2-treated HEK293 cells (1 mM) were injected into a deubiquitinating assay buffer containing 0.5% NP40 and Ub-AFC. The fluorescence intensity was recorded immediately after the addition of the cells. (b) PCNA ubiquitination is induced by H2O2treatment. HEK293 cells were treated with 1 mM H2O2for the indicated time periods. Cells were lysed directly in the Laemmli buffer before immunoblotting (IB) analyses. (c) A DUB inhibitor induces PCNA ubiquitination. HEK293 cells were treated with 20 μM PR-619 for the indicated time periods. A fraction of the cells were lysed in the Laemmli buffer for IB (top panel). The DUB activities in the remaining cells were also determined (bottom panel). (d) DNA damage and DUB inhibition synergistically induce PCNA monoubiquitination. The number indicates the intensity of the Ub-PCNA bands. (e) Quantification of ubiquitinated PCNA as per cent of total PCNA in untreated cells or cells treated with the indicated chemicals for 1 h (MMS 1 mM; PR-619, 20 μM; error bars represent means of two independent experiments). (f) H2O2wash-out causes deubiquitination of PCNA. Cells treated with H2O2(0.5 mM, 15 min) were incubated in a fresh medium in the absence or presence of the DUB inhibitor PR-619. Whole-cell extracts were analysed by IB. (g) Deubiquitination of PCNA after H2O2removal requires USP1. As inf, except that cells treated with the indicated knockdown constructs were used. (h,i) H2O2-treated nuclear extract (NE) fails to cleave ubiquitin from PCNAin vitro. (h)In vitroubiquitinated PCNA was incubated with NE, H2O2-treated NE or NE with the DUB inhibitor ubiquitin aldehyde (Ub-Al). (i)In vitroubiquitinated PCNA was incubated with NE or H2O2-treated NE for the indicated time points. Figure 6: DUB inhibition in oxidative-stressed cells facilitates PCNA ubiquitination. ( a ) The kinetics of DUB inhibition by H 2 O 2 . H 2 O 2 -treated HEK293 cells (1 mM) were injected into a deubiquitinating assay buffer containing 0.5% NP40 and Ub-AFC. The fluorescence intensity was recorded immediately after the addition of the cells. ( b ) PCNA ubiquitination is induced by H 2 O 2 treatment. HEK293 cells were treated with 1 mM H 2 O 2 for the indicated time periods. Cells were lysed directly in the Laemmli buffer before immunoblotting (IB) analyses. ( c ) A DUB inhibitor induces PCNA ubiquitination. HEK293 cells were treated with 20 μM PR-619 for the indicated time periods. A fraction of the cells were lysed in the Laemmli buffer for IB (top panel). The DUB activities in the remaining cells were also determined (bottom panel). ( d ) DNA damage and DUB inhibition synergistically induce PCNA monoubiquitination. The number indicates the intensity of the Ub-PCNA bands. ( e ) Quantification of ubiquitinated PCNA as per cent of total PCNA in untreated cells or cells treated with the indicated chemicals for 1 h (MMS 1 mM; PR-619, 20 μM; error bars represent means of two independent experiments). ( f ) H 2 O 2 wash-out causes deubiquitination of PCNA. Cells treated with H 2 O 2 (0.5 mM, 15 min) were incubated in a fresh medium in the absence or presence of the DUB inhibitor PR-619. Whole-cell extracts were analysed by IB. ( g ) Deubiquitination of PCNA after H 2 O 2 removal requires USP1. As in f , except that cells treated with the indicated knockdown constructs were used. ( h , i ) H 2 O 2 -treated nuclear extract (NE) fails to cleave ubiquitin from PCNA in vitro . ( h ) In vitro ubiquitinated PCNA was incubated with NE, H 2 O 2 -treated NE or NE with the DUB inhibitor ubiquitin aldehyde (Ub-Al). ( i ) In vitro ubiquitinated PCNA was incubated with NE or H 2 O 2 -treated NE for the indicated time points. Full size image Because the kinetics of PCNA ubiquitination resemble those of DUB inhibition in H 2 O 2 -treated cells and also because H 2 O 2 does not significantly affect the activities of the ubiquitin conjugating machineries ( Supplementary Fig. S8c ), we reasoned that PCNA ubiquitination upon H 2 O 2 treatment might result from DUB inhibition. In support of this notion, incubation of cells with the DUB inhibitor PR-619 was sufficient to induce PCNA mono-ubiquitination rapidly even in the absence of any DNA damages ( Fig. 6c ). Moreover, the DNA damaging agent MMS, which does not inhibit DUBs, only induced PCNA ubiquitination inefficiently, but co-treatment of cells with PR-619 and MMS synergistically induced PCNA ubiquitination ( Fig. 6d ). To further test the role of DUB inhibition in PCNA ubiquitination, we performed a H 2 O 2 wash-out experiment in which cells exposed to H 2 O 2 were further incubated in a H 2 O 2 -free medium. Over time, the levels of ubiquitinated PCNA in cells were reduced ( Fig. 6f ). The loss of ubiquitinated PCNA after removal of H 2 O 2 was strongly inhibited by either the DUB inhibitor PR-619 ( Fig. 6f ) or knockdown of USP1 ( Fig. 6g ), a DUB previously implicated in regulating PCNA ubiquitination [8] . Collectively, these results indicate that inhibition of DUBs (USP1 in particularly) in cells encountering acute oxidative stress accounts for the rapid accumulation of monoubiquitinated PCNA. We next wished to recapitulate the redox-dependent regulation of PCNA ubiquitination in vitro . We found that incubation of in vitro -synthesized ubiquitinated PCNA ( Supplementary Fig. S8d ) with a nuclear extract (NE) resulted in the loss of ubiquitinated PCNA that could be blocked by the DUB-specific inhibitor ubiquitin aldehyde, suggesting the presence of a DUB activity in NE that efficiently removes ubiquitin from PCNA ( Fig. 6h ). Treatment of NEs in vitro with H 2 O 2 strongly inhibited this activity as ubiquitinated PCNA was completely stable when incubated with H 2 O 2 -treated NE ( Fig. 6h ). These results demonstrate a redox regulation of DUBs in NE that directly controls ubiquitination of PCNA. H 2 O 2 inhibits USP1 when the cofactor UAF1 is present Our results so far showed that inhibition of USP1 allows PCNA to undergo ubiquitination in oxidatively stressed cells. However, our initial study suggested that purified USP1 alone is not activated by DTT ( Table 1 ). One explanation for this paradox is that the activation of USP1 requires its cofactor(s), as demonstrated previously [40] . Thus, the redox-dependent regulation may only affect USP1 when it is in complex with the activator UAF1. To test this possibility, we purified the UAF1–USP1 complex under reducing conditions ( Fig. 7a ). Using the Ub-AFC assay, we demonstrated that this complex was indeed active in vitro ( Fig. 7b ), but the activity was strongly inhibited by H 2 O 2 in a reversible manner ( Fig. 7b ). H 2 O 2 does not affect the interaction of USP1 with UAF1 ( Supplementary Fig. S9 ), suggesting that the inhibition is likely caused by oxidation of USP1 active site. 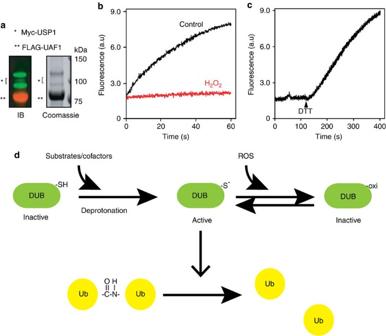Figure 7: Oxidative stress inhibits USP1 in complex with UAF1. (a) The purified USP1–UAF1 complex. (b) The activity of the USP1–UAF1 complex is inhibited by H2O2. Where indicated, the USP1–UAF1 complex was treated with H2O2(0.5 mM, 5 min). The DUB activities were determined by the Ub-AFC assay. (c) USP1 inhibition by H2O2is reversed by DTT. The activity of the H2O2-treated USP1–UAF1 complex was measured. Where indicated, DTT was added to the reaction. (d) A model depicting the redox regulation of DUBs. Figure 7: Oxidative stress inhibits USP1 in complex with UAF1. ( a ) The purified USP1–UAF1 complex. ( b ) The activity of the USP1–UAF1 complex is inhibited by H 2 O 2 . Where indicated, the USP1–UAF1 complex was treated with H 2 O 2 (0.5 mM, 5 min). The DUB activities were determined by the Ub-AFC assay. ( c ) USP1 inhibition by H 2 O 2 is reversed by DTT. The activity of the H 2 O 2 -treated USP1–UAF1 complex was measured. Where indicated, DTT was added to the reaction. ( d ) A model depicting the redox regulation of DUBs. Full size image In this study, we demonstrate a redox-dependent regulatory mechanism that controls DUB activities in vitro and in cells ( Fig. 7d ). We show many DUBs upon activation are prone to oxidation due to the presence of a deprotonated cysteine at the active site, suggesting that the chemistry of deubiquitination inevitably imposes risks of oxidative damages on DUBs. Therefore, it is conceivable that DUBs are under evolutionary pressure to operate in a parsimonious manner (see below), which would reduce undesired damage by oxidation. Consistent with this notion, we show that although cysteine-based DUBs share a similar catalytic triad, ∼ 40% of the DUBs analysed do not contain any activity even in the reduced form. These enzymes appear to be controlled by additional factors or posttranslational modifications, as demonstrated previously [29] , [31] , [40] , [41] , [42] , [43] , [44] , [45] , [46] , [47] . Therefore, redox regulation is only applicable when these DUBs are in complex with their cofactors, as exemplified by USP1. Although ROS can inhibit many cysteine proteases, it is noteworthy that not every cysteine protease family is equally sensitive to ROS. For example, caspases and calpain can both be activated by oxidative stress to mediate apoptosis [48] , [49] . In this regard, although our studies show that ROS affects many DUBs, we cannot exclude the possibility that a few DUBs may have evolved mechanisms that prevent ROS-mediated oxidation. Several aspects of the redox-dependent DUB regulation are worth noting. First, the inhibition of DUBs by ROS is reversible even after prolonged exposure to H 2 O 2 . Even in the presence of H 2 O 2 , the DUB activity in cells displays a time-dependent partial recovery. This recovery is likely due to the activation of many anti-oxidative genes that reduces ROS levels. It is also interesting to consider the chemistry of cysteine oxidation. In stressed cells, cysteine oxidation can occur when its sulfhydryl group is converted to sulphenic acid (-SOH), which can be further oxidized into a disulphide or a sulphenyl-amide form. Sulphenic acid can also be converted into sulphinic acid (-SO 2 H) or sulphonic acid (-SO 3 H). Only the disulphide, sulphenyl-amide and sulphenic acid forms can be reduced by a thiol-reducing agent [50] . For USP19, only a small fraction of the enzyme forms intermolecular disulphide upon treatment with H 2 O 2 , and no sulphenic group could be captured and detected by dimedone (Lee J., unpublished results). Thus, the majority of the oxidized cysteine in USP19 is likely in the sulphenyl-amide form in which the side chain of the cysteine reacts with a nitrogen atom in a proximal amino acid, as demonstrated for the PTPs [22] . This is indeed confirmed by mass spectrometry. The redox regulation of DUBs displays some similarity to that of PTPs with the exception that the inhibition of DUBs by ROS occurs in a highly regulated manner as the activities of many DUBs are regulated by cofactors/substrates. Given the broad interplays between DUBs and various signalling processes, it is tempting to speculate that reversible inactivation of DUBs and PTPs may act in parallel in cells encountering oxidative stress to control signal transduction and to promote cellular adaptation to oxidative damages. Oxidative stress can inflict significant damages to DNA including strand breaks and base modifications. A major protein coordinator of the eukaryotic DNA damage tolerance programme is the replication clamp PCNA. PCNA can be modified with mono-ubiquitin, ubiquitin chains or the small ubiquitin-like modifier in response to DNA damage [39] . Different types of PCNA modification are thought to govern a switch between a DNA repair pathway and a damage tolerance programme. Monoubiquitinated PCNA recruits the low-fidelity DNA polymerases, maintaining DNA replication despite the lesions [51] , [52] . The initiation of this so-called TLS programme allows cells to proliferate at the expense of genome stability under oxidative stress conditions, a feature particularly critical for the growth of cancer cells. The mechanism that regulates PCNA ubiquitination in cells encountering oxidative stress has been unclear. Our study reveals an important role of DUB inhibition in this process. In normal cells, USP1 serves as a ‘brake’ that keeps PCNA in the unmodified form. Oxidative stress not only induces DNA damages, but also inactivates USP1, allowing ubiquitinated PCNA to rapidly accumulate in cells to launch the TLS programme. Consistent with this notion, a recent study showed that ultraviolet treatment also causes rapid accumulation of mono-ubiquitinated PCNA as a result of inactivation of USP1 by ultraviolet -induced autocleavage, causing genome instability [8] . It is noteworthy that ultraviolet-induced inactivation of USP1 is mechanistically distinct from ROS-mediated DUB inactivation. While our paper was under review, Cotto-Rios et al . reported similar findings that inhibition of USP1 by oxidative stress is causal to mono-ubiquitination of PCNA [53] . Based on these results, we propose that DUB inhibition contributes to increased genome instability associated with oxidative stress by allowing PCNA mono-ubiquitination to occur. Although the current study emphasizes on the role of DUBs in regulating a DNA damage-tolerance programme coordinated by ubiquitinated PCNA, oxidative stress-induced DUB inhibition can occur globally, thus potentially impacting many other substrates in cells. Inhibition of DUBs by ROS takes place in a short-time frame, in which many redox-regulated signalling processes are elicited [33] . Therefore, reversible inactivation of DUBs under acute oxidative stress conditions may also regulate signalling outputs by altering the ubiquitination status of many signalling molecules. Primers The following primers were used for plasmid construction: USP19 WT Forward, 5′-AAACGCGTCGACCATGTCTGGCGGGGCCAGTG-3′ Reverse, 5′-ATAAGAAGGCGGCCGCTTATCTCCAGCGACTCTGGGATAC-3′ USP19CD Forward, 5′-AAACGCGTCGACCCCAGGCTTCACTGGCCTGTC-3′ Reverse, 5′-ATAAGAAGGCGGCCGCTTACCGGAGGCAGCCCTCATCTG-3′ USP8CD Forward, 5′-AAACGCGTCGACCCCAACAGTAACTCCAACAG-3′ Reverse, 5′- ATAAGAAGGCGGCCGCTTATCCCAATGAAGTATAAAAG-3′ Plasmids and other reagents The HEK293, HepG2 and RAW264.7 cell lines were obtained from American Type Culture Collection and cultured under standard conditions in DMEM medium. Plasmids expressing FLAG-tagged DUBs were provided generously by J.W. Harper through Addgene (Cambridge, MA). The USP19 complementary DNA was further subcloned by ligating the PCR-amplified cDNA fragments into the Sal I and Not I sites of the pRK-FLAG vector [54] . To express the catalytic domain of USP8 and USP19, we amplified the predicted DNA fragments encoding the USP8 CD (residue 734–1,110) and USP19 CD (residue 494–1,290) and cloned these DNA fragment between the Sal I and Not I sites of the pRK-FLAG vector. Each catalytic inactive CD mutant was generated by site-directed mutagenesis using standard procedure. TransIT-293 (Mirus) was used for plasmid transfection. Antibodies used are FLAG (M2, Sigma), Biotin (Rockland), PCNA (PC10, Santa Cruz) and Ubiquitin (P4D1, Santa Cruz). UBE1, Rad6B and Ub-AFC were purchased from Boston Biochem. CM-DCFDA was purchased from Invitrogen. USP4, Rad18 and PCNA were purchased from Origene. Ubiquitin and NEM were purchased from Sigma. Maleimide-Biotin was purchased from Thermo Scientific. PR-619 was purchased from LifeSensors. Immunoblotting Cells were lysed in the NP40 lysis buffer containing 50 mM Tris–HCl pH 7.4, 150 mM sodium chloride, 2 mM magnesium chloride, 0.5% NP40 and a protease inhibitor cocktail [55] . Cell extracts were subject to centrifugation to remove insoluble materials. Immunoblotting was performed according to the standard protocol. Fluorescence-labelled secondary antibodies were used for detection. The fluorescent bands were imaged and quantified by a LI-COR Odyssey infrared imager using the software provided by the manufacture. Protein purification To purify deubiquitinating enzymes, HEK293 cells grown in 10-cm culture dishes were transfected with the individual DUB-expressing plasmid. Cells were propagated for 72 h before lysis in a buffer containing 1% 3-[(3-Cholamidopropyl)dimethylammonio]-1-propanesulfonate (CHAPS), 1% Triton X-100, 50 mM Tris–HCl pH 7.4, 150 mM sodium chloride, 2 mM magnesium chloride, 1 mM EDTA and a protease inhibitor cocktail. The cleared cell extract was incubated with FLAG-agarose beads (Sigma) and the bound materials were extensively washed with a buffer containing 0.1% CHAPS, 0.1% Triton X-100, 50 mM Tris–HCl pH 7.4, 150 mM sodium chloride, 2 mM magnesium chloride, 1 mM EDTA. The bound materials were eluted using 0.2 mg ml −1 FLAG peptide (Sigma) in 25 mM HEPES pH 7.2, 115 mM potassium acetate, 5 mM sodium acetate, 2.5 mM magnesium chloride. For purifications under the reducing condition, the lysis and wash buffers also contain 1.0 mM DTT and the elution buffer contains 0.5 mM DTT. Quantitative immunoblotting was performed using known concentrations of FLAG-tagged ubiquitin or BSA as a reference to determine the concentrations for the purified proteins. ROS measurement To determine the levels of H 2 O 2 in cells, cells were treated with the CM-DCFDA dye (10 μM) and the fluorescence intensity was determined by the Cytomics FC 500MPL Flow Cytometry System (Beckman Coulter) following the manufacture’s instruction. Biotin labelling and HA-Ub-VS Labelling experiments Cells transfected with the indicated DUB-expressing plasmids were treated with or without 1 mM H 2 O 2 for 5 min and lysed in the labelling buffer containing 10 mM NEM, 50 mM Tris–HCl pH 7.0, 120 mM sodium chloride, 0.5 mM EDTA, 0.5% NP40 and a protease inhibitor cocktail. The cleared cell extract was incubated with 1% SDS to allow modifying all the cysteine residues except for the oxidized one by NEM at room temperature for 2 h. The cell extract was diluted with 50 mM Tris-HCl pH 7.0, 120 mM sodium chloride, 0.5 mM EDTA to adjust the concentration of SDS to 0.1% and FLAG-tagged DUBs were immunoprecipitated by FLAG-agarose beads. The bound DUB enzyme was treated with 10 mM DTT for 10 min to reduce the oxidized cysteine residue. The reduced DUB enzyme on the beads was labelled with 0.2 mM maleimide-biotin in 50 mM Tris–HCl pH 7.0, 120 mM sodium chloride, 0.5 mM EDTA for 1 h. The bound materials were eluted using the SDS sample buffer and analysed by immunoblotting. For labelling DUBs by Ub-VS, cells washed with PBS were treated with a labelling buffer containing 0.5% NP40 and HA-Ub-VS (2 μM). Cells were incubated at 37 °C for 10 min before immunoblotting analysis. For the mass spectrometry experiments, the band corresponding to oxidized USP19 was digested with trypsin and extracted. Precursor ion (1,211.89 m / z ) was isolated and fragmented in a Velos Orbitrap (Thermo). In vitro PCNA ubiquitination and deubiquitination For in vitro ubiquitination of PCNA, purified PCNA (2 μM) was incubated with 100 nM UBE1, 2 μM RAD6B, 2 μM RAD18, 12 μM ubiquitin in a buffer containing 25 mM Tris-HCl pH 7.4, 2 mM magnesium chloride, 1 mM DTT and 2 mM ATP at 37 °C for 14 h. For deubiquitination of PCNA in vitro , NE was prepared as follows: cells were collected and washed with ice-cold PBS twice. Cells were then resuspended in a hypotonic buffer containing 20 mM HEPES pH 7.2, 10 mM potassium chloride, 1 mM magnesium chloride, 1 mM DTT and a protease inhibitor cocktail on ice for 10 min and were broken using a Dounce homogenizer. The nuclei of the cells were obtained by centrifugation at 1,000 g for 10 min at 4 °C. The nucleus pellet fraction was washed with a hypotonic buffer and resuspended in the high salt extraction buffer containing 20 mM Tris-HCl pH 8.0, 450 mM sodium chloride, 2 mM magnesium chloride, 0.2 mM EDTA and a protease inhibitor cocktail. The sample was subject to centrifugation at 16,100 g for 5 min at 4 °C and the supernatant fraction was collected as NE after centrifugation. To monitor PCNA deubiquitination in the presence of NE, we repurified FLAG-tagged PCNA after it has been ubiquitinated in vitro . The beads containing ubiquitinated PCNA were incubated with NE either untreated or pretreated with 1 mM H 2 O 2 , and the samples were analysed by immunoblotting. In vitro DUB assays The activity of purified DUBs was determined by detecting the increase in fluorescence upon cleavage of Ub-AFC (Boston Biochem). Unless specified in the figure legends, purified DUBs ( ∼ 200 nM) were added individually to 200 μl deubiquitinating assay buffer (50 mM Tris–HCl pH 7.4, 20 mM potassium chloride, 5 mM magnesium chloride including 0.5 μM Ub-AFC), and incubated at 37 °C. The fluorescence intensity was measured using an Aminco Bowman Luminescence spectrometer with excitation and emission wavelengths set at 400 and 505 nm, respectively. To measure the in vivo DUB activity (experiments in Fig. 6b ), the same number of cells ( ∼ 3,000) after various treatments was directly added to the deubiquitinating assay buffer that also contains 0.5% NP40 and the cleavage of Ub-AFC was immediately monitored for 2 min. In some experiments (experiments in Fig. 4 ), cells were lysed in a lysis buffer containing 50 mM Tris–HCl pH 7.4, 150 mM sodium chloride, 2 mM magnesium chloride, 0.5% NP40 and a protease inhibitor cocktail, and the DUB activity in whole-cell extract was measured within 5 min of cell lysis. Data obtained were plotted and analysed using Kaleidagraph v4.0 (Synergy Software). In some experiments, we used K48-linked di-ubiquitin as a model substrate to determine DUB activity. In this case, 1 μg di-ubiquitin was incubated with ∼ 500 nM DUB in 20 μl DUB assay buffer. The cleavage of di-ubiquitin was monitored by SDS–PAGE gel followed by Coomassie blue staining. How to cite this article: Lee, J.-G. et al . Reversible inactivation of deubiquitinases by reactive oxygen species in vitro and in cells. Nat. Commun. 4:1568 doi: 10.1038/ncomms2532 (2013).